Synthetic ligands for PreQ1riboswitches provide structural and mechanistic insights into targeting RNA tertiary structure Riboswitches are naturally occurring RNA aptamers that regulate gene expression by binding to specific small molecules. Riboswitches control the expression of essential bacterial genes and are important models for RNA-small molecule recognition. Here, we report the discovery of a class of synthetic small molecules that bind to PreQ 1 riboswitch aptamers. These molecules bind specifically and reversibly to the aptamers with high affinity and induce a conformational change. Furthermore, the ligands modulate riboswitch activity through transcriptional termination despite no obvious chemical similarity to the cognate ligand. X-ray crystallographic studies reveal that the ligands share a binding site with the cognate ligand but make different contacts. Finally, alteration of the chemical structure of the ligand causes changes in the mode of RNA binding and affects regulatory function. Thus, target- and structure-based approaches can be used to identify and understand the mechanism of synthetic ligands that bind to and regulate complex, folded RNAs. An explosion of interest in RNA biology in recent years has revealed a multitude of new regulatory functions for noncoding RNA [1] , [2] . Many noncoding RNAs regulate gene expression or protein function and are often dysregulated in cases of infectious disease or cancer [3] , [4] . The observation that regulatory, noncoding RNAs can directly influence disease states [5] has led to the suggestion that such RNAs could be suitable as targets for small molecules [6] , [7] , [8] . Thus, the goal of developing RNA-binding small molecules as both therapeutics and chemical probes is an area of increasing interest. However, the discovery of molecules that bind to RNA with good affinity and specificity is a major challenge owing to RNA’s highly flexible, dynamic structure and largely solvent-exposed binding pockets, in addition to the fact that many RNAs are actively unfolded in the cell [9] . Further, understanding the function of noncoding RNA has proven highly challenging in many cases [10] . Although it is now routine to utilize structure to rationalize the function of protein-binding small molecules, high-resolution structures of RNA are often difficult to determine. The challenge in characterizing the specific contacts small molecules make with RNAs is often a substantial impediment to understanding and developing small molecule probes of RNA. One class of regulatory, noncoding RNAs where major advances in structure determination have been seen is riboswitches. Riboswitches are structured RNA elements that occur in the untranslated regions of mRNA, most often in bacteria [11] . Riboswitches act as regulators of gene expression through recognition of a small-molecule ligand that induces a conformational change in the RNA, thereby regulating downstream gene expression [12] . Riboswitches often recognize ligands related to the function of the associated gene product [13] and, in some examples, the ligand can be a product of the biosynthetic pathway regulated by the riboswitch. Molecules recognized can range from nucleobases, cofactors, and amino acids to metal ions [13] . These structured RNA elements have two domains, an aptamer domain that recognizes the cognate ligand through specific interactions, and an expression platform that changes conformation upon binding to modulate gene expression [12] . Riboswitch-mediated gene regulation can occur at either the transcriptional or translational level. For transcriptional riboswitches, cognate ligand binding usually promotes an RNA conformation that contains a terminator helix that triggers dissociation of RNA polymerase and leads to transcription termination upstream of the coding sequence. In the absence of the ligand, the RNA folds into an alternate antiterminator, therefore, allowing transcription of the downstream gene. In translational riboswitches, ligand binding causes a conformational change that produces a helix that occludes the Shine-Dalgarno sequence and prevents ribosomal binding. In the absence of the ligand, an alternate structure forms, increasing the availability of the ribosomal binding region and facilitating translation initiation. The ability of riboswitches to control essential bacterial genes has stimulated their evaluation as antibacterial targets. Furthermore, riboswitches also serve as important model systems for highly specific RNA-small molecule interactions [14] , [15] , [16] , [17] , [18] , [19] , [20] , [21] , [22] . The PreQ 1 riboswitch governs the expression of genes responsible for the biosynthesis of queuosine (Q) [23] . The riboswitch regulates downstream gene expression in response to its cognate ligand PreQ 1 (7-aminomethyl-7-deazaguanine). PreQ 1 is a modified, guanine-derived nucleobase that is incorporated into tRNAs at the wobble position, where it is further altered to produce Q [24] . The role of Q is linked to the preservation of translational fidelity and aids reading of degenerate codons. Further, removal of enzymes involved in Q biosynthesis results in multiple phenotypic defects in a variety of organisms [25] , [26] . This pathway is thought to be essential for bacterial virulence in some cases [27] . Many organisms contain PreQ 1 riboswitches, and to date, three distinct PreQ 1 riboswitch classes have been discovered that differ in both sequence and mechanism [23] . Importantly, class I PreQ 1 (PreQ 1 -I) riboswitches, such as that found in Bacillus subtilis ( Bs ), are among the smallest known riboswitches, with the Bs riboswitch having a minimal aptamer domain of just 34 nucleotides (nt). In Bs , the PreQ 1 riboswitch regulates the queCDEF operon that is involved in Q biosynthesis. Upon ligand binding, the Bs PreQ 1 riboswitch folds into an H-type pseudoknot [28] causing a conformational change that induces a terminator hairpin and downregulates transcription. Similarly, the PreQ 1 -I riboswitch from Thermoanaerobacter tengcongensis ( Tt ) also adopts an H-type pseudoknot structure [29] in the ligand-bound state. In contrast, the Tt riboswitch regulates expression of a PreQ 1 transporter [30] and does so via translational inhibition by a conformational change that sequesters the Shine-Dalgarno sequence. The small and well-characterized aptamer domains of the PreQ 1 riboswitches from Bs and Tt make them ideal model systems for assessing the ability to target riboswitches with synthetic small molecules to regulate downstream gene expression [31] . In this study, we report the discovery of a new class of synthetic small molecules that bind directly to PreQ 1 riboswitches. We performed a small molecule microarray (SMM) screen on the aptamer domain of the PreQ 1 riboswitch found in Bs . Hit compounds that showed selective binding to the riboswitch over other RNAs were validated through a series of biophysical experiments. One hit compound from this screen exhibits a dissociation constant of ~ 500 n m to the Bs PreQ 1 aptamer by multiple orthogonal fluorescence titrations. Further, in-line probing suggests that the synthetic ligand induces a riboswitch conformation that is different from that of the cognate ligand-bound form. The compound is also shown to bind the structurally similar, but functionally distinct Tt PreQ 1 riboswitch. Co-crystal structures with this aptamer show that the compound binds in the PreQ 1 -binding site but makes key interactions with conserved nucleotides that are different from those of the cognate ligand. Importantly, in vitro transcription termination assays demonstrate that the small molecule is capable of regulating riboswitch function upon binding. Structure-guided alteration of the chemical structure of the ligand impacts both the mode of binding and activity of the ligands. The co-crystal structures will further be used for developing additional compounds that target the PreQ 1 riboswitch and the Q biosynthetic pathway. SMM screening of a PreQ 1 riboswitch aptamer To identify drug-like small molecules that bind to the PreQ 1 riboswitch, we used a SMM-screening strategy [32] , [33] , [34] , [35] , [36] , [37] , [38] , [39] , [40] . In this approach, small molecules are spatially arrayed and covalently linked to a glass surface. Next, a fluorescently tagged RNA of interest is incubated with the arrays. Slides are washed, imaged, and the fluorescence intensity is measured for each location on the array. For each compound (printed in duplicate), a composite Z-score is generated, reflecting the increase in fluorescence upon addition of labeled RNA. In parallel, other RNAs may be counter screened to evaluate selectivity and prioritize hit compounds that arise from the screen. Toward this end, we designed a 5′-Cy5-labeled RNA consisting of the 34-nt aptamer domain of the PreQ 1 riboswitch from Bs (5ʹ-Cy5- Bs PreQ 1 -RS, Fig. 1A ) [30] . Once purity was confirmed by gel electrophoresis, the RNA was annealed and incubated on SMM slides to perform the screen. 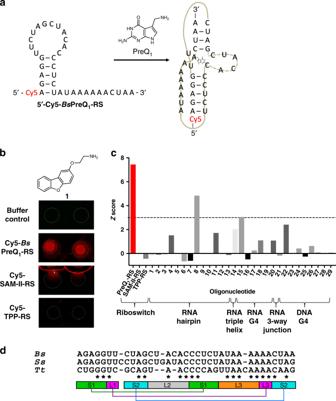Fig. 1 Small molecule microarray screening.aSequence of the Cy5-labeled aptamer domain of theBsPreQ1riboswitch (5′-Cy5-BsPreQ1-RS) used for SMM screening. The conformational change induced by PreQ1binding is also shown.bSMM images for the hit compound1(compound is printed in duplicate). Spot diameter (white circle) is 150 µm.cSelectivity of the hit compound across various oligonucleotides screened using the SMM platform (Supplementary Table2) as measured by composite Z-score. Horizontal line corresponds to a “hit” cutoff of 3.dSequence alignment ofBs,Ss, andTtPreQ1riboswitch aptamers. Conserved nucleotides are marked by asterisks. Secondary structure of the class I PreQ1riboswitch aptamers is below the alignment and base-pairing interactions are indicated by colored bars In parallel, we also screened analogous 5′-Cy5-labeled constructs consisting of aptamer domains from S -adenosylmethionine (SAM-II) [41] and thiamine pyrophosphate (TPP) [42] riboswitches (Supplementary Table 1 ). Each of these three aptamer domains are known to recognize different biologically active ligands and have well defined, complex three-dimensional structures, making them suitable controls for selectivity. 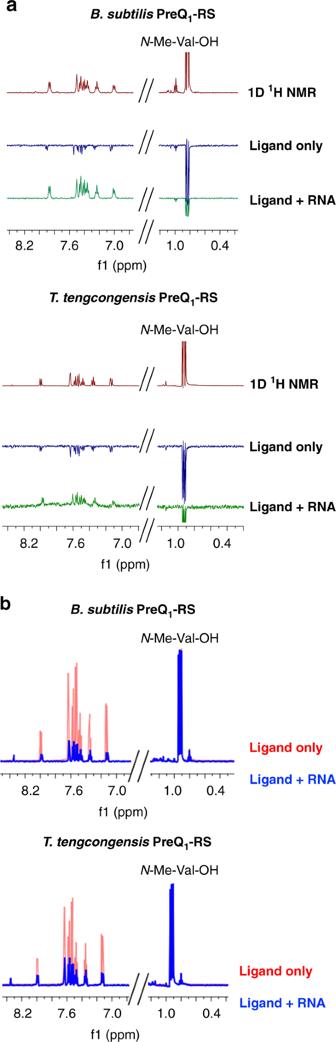Fig. 2 NMR validation of hit compound1.a1H NMR of1andN-methyl-l-valine (non-binding control) (Top, red spectrum), WaterLOGSY NMR of1andN-methyl-l-valine in the absence (middle, blue spectrum) and presence (bottom, green spectrum) of either theBsorTtPreQ1riboswitch aptamer.bCPMG of1andN-methyl-l-valine in the absence (red) and presence (blue) of either theBsorTtPreQ1riboswitch aptamer To further measure selectivity, the Z-score for each compound is compared across many different SMM screens (in this case 29 different oligonucleotides, Supplementary Table 2 ). We identified 243 hits from a collection of 26,227 compounds screened in the SMM, for an initial hit rate of 0.93%. 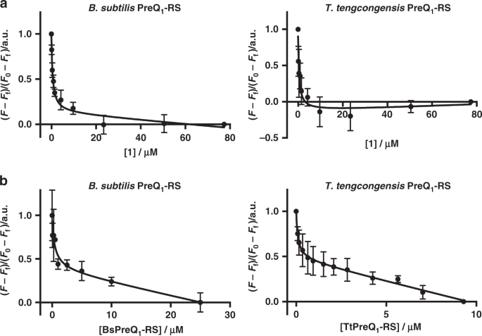Fig. 3 Affinity of1for PreQ1-RS aptamers.aFluorescence intensity assay of 5′-Cy5-labeledBsPreQ1-RS or 5′-AlexaFluor 647-labeledTtPreQ1-RS RNA in the presence of increasing concentration of1.bInherent fluorescence titration of1with increasing concentration of unlabeledBsPreQ1-RS orTtPreQ1-RS RNA. Error bars indicate the standard deviation determined from three independent measurements. Source data are provided as a Source Data file After ruling out compounds that bound promiscuously to other riboswitches or other RNAs and DNAs previously screened against the library, we generated a list of 86 candidate compounds for further study (Supplementary Table 3 ). The TPP and SAM-II riboswitches had slightly fewer numbers of “selective” hits, with rates of 51 hits (0.19%) and 61 hits (0.23%), respectively. 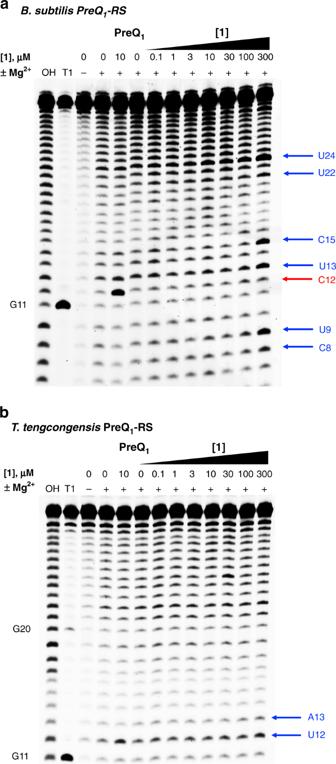Fig. 4 Ligand-induced conformational changes. In-line probing ofa5′-AlexaFluor 647-labeledBsPreQ1-RS RNA andb5′-AlexaFluor 647-labeledTtPreQ1-RS RNA after treatment with1at increasing concentrations or a DMSO control in the absence (–) or presence (+) of 1 mmMgCl2. Treatment with PreQ1at a concentration of 10 μmis used as a positive control. OH and T1 are a partial alkaline hydrolysis ladder and ribonuclease T1 digestion, respectively. Arrows designate nucleotide positions where the cleavage efficiency was significantly altered by compound treatment (blue) or preQ1treatment (red) Twenty hits identified as selective for the PreQ 1 aptamer were purchased for further analysis (Supplementary Table 4 and Supplementary Fig. 1 ). As a representative example, direct binding on SMM slides (Fig. 1B ) and selectivity data (Fig. 1C ) are shown for compound 1 . Fig. 1 Small molecule microarray screening. a Sequence of the Cy5-labeled aptamer domain of the Bs PreQ 1 riboswitch (5′-Cy5- Bs PreQ 1 -RS) used for SMM screening. The conformational change induced by PreQ 1 binding is also shown. b SMM images for the hit compound 1 (compound is printed in duplicate). Spot diameter (white circle) is 150 µm. c Selectivity of the hit compound across various oligonucleotides screened using the SMM platform (Supplementary Table 2 ) as measured by composite Z-score. Horizontal line corresponds to a “hit” cutoff of 3. d Sequence alignment of Bs , Ss , and Tt PreQ 1 riboswitch aptamers. Conserved nucleotides are marked by asterisks. Secondary structure of the class I PreQ 1 riboswitch aptamers is below the alignment and base-pairing interactions are indicated by colored bars Full size image Ligand observed NMR validates binding Each of the purchased compounds was evaluated using Water-Ligand Observed via Gradient Spectroscopy (WaterLOGSY) NMR [43] . In this experiment, each compound was subjected to a standard 1 H NMR pulse sequence (to assess solubility in aqueous buffer), WaterLOGSY without RNA (to assess aggregation), and WaterLOGSY in the presence of unlabeled Bs PreQ 1 -RS RNA (to assess binding to the riboswitch aptamer) (Fig. 2A ). For compounds that bind directly to the RNA, peaks phase positively only in the presence of RNA. In contrast, aggregating compounds phase positively even in the absence of RNA. Peaks for compounds that are soluble but do not bind to the RNA are phased negatively in both cases (as can be seen with N -methyl- l -valine, included here as a convenient internal, non-binding control). From these experiments, we identified five compounds with suitable solubility and RNA binding in the solution phase. We also evaluated binding of each compound against 31 different structured RNAs and DNAs from previous SMM screens, where compound 1 was found to have the best profile of selective binding (Fig. 1C ). Fig. 2 NMR validation of hit compound 1 . a 1 H NMR of 1 and N -methyl- l -valine (non-binding control) (Top, red spectrum), WaterLOGSY NMR of 1 and N -methyl- l -valine in the absence (middle, blue spectrum) and presence (bottom, green spectrum) of either the Bs or Tt PreQ 1 riboswitch aptamer. b CPMG of 1 and N -methyl- l -valine in the absence (red) and presence (blue) of either the Bs or Tt PreQ 1 riboswitch aptamer Full size image To further validate these results, we also evaluated 1 by WaterLOGSY NMR with a second PreQ 1 riboswitch aptamer domain from Tt (unlabeled Tt PreQ 1 -RS, Supplementary Table 1 ) [29] . Although divergent in sequence and genetic control mechanism [44] , this riboswitch also recognizes the same cognate ligand and has a mostly conserved binding site. Gratifyingly, 1 also bound directly to the Tt PreQ 1 aptamer domain by WaterLOGSY (Fig. 2A ). In addition to WaterLOGSY experiments, we evaluated the behavior of 1 in Carr-Purcell-Meiboom-Gill (CPMG) 1 H NMR experiments, which can be used to observe alterations in T 2 relaxation times of small molecules that bind large molecules in solution (with binding shortening relaxation time) [45] , [46] . Here, 1 was subjected to a CPMG pulse sequence in the absence and presence of both the Bs and Tt aptamers used in the WaterLOGSY experiments. In both cases, substantial peak attenuation of 1 with no attenuation of the control was observed in the presence of RNA, indicating shortening of the T 2 relaxation time of protons in 1 (Fig. 2B ). Thus, CPMG experiments further validate the binding of 1 to both aptamers. Because the two aptamers have conserved binding sites but diverge moderately in structure, this suggested that 1 could potentially share a binding site with the cognate ligand. Fluorescence titrations demonstrate submicromolar binding To estimate the affinity of 1 to the PreQ 1 riboswitch aptamer domain, we used orthogonal fluorescence titrations. First, we measured changes in fluorescence of the Cy5-labeled Bs aptamer domain construct used for SMM screening (5ʹ-Cy5- Bs PreQ 1 -RS) as a function of compound concentration. In parallel, we evaluated effects on an AlexaFluor 647-labeled Tt aptamer domain construct (5ʹ-AF647- Tt PreQ 1 -RS, Supplementary Table 1 ) to both measure affinity and further rule out effects associated with the fluorophore (Fig. 3A ). In the case of the Bs aptamer, we measured an apparent dissociation constant ( K D ) of 534 ± 123 n m for 1 . Similarly, 1 had a K D of 457 ± 202 n m for the Tt aptamer domain. For comparison, we also measured the affinity of PreQ 1 itself in this assay. The affinity of PreQ 1 for the Bs aptamer was 4.1 ± 0.6 nM, and for the Tt aptamer it was 2.8 ± 0.4 n m (Supplementary Fig. 2 ). This is in good agreement with literature values measured by other methods [29] , [30] , [44] . Owing to the presence of a conjugated π-electron system, we evaluated 1 for inherent fluorescence and found that 1 was fluorescent, with λ ex = 300 nm and λ em = 340 nm. Thus, by holding the concentration of 1 constant and titrating in increasing quantities of unlabeled riboswitch aptamers, we could measure K D values by observing changes in fluorescence as a function of RNA concentration (Fig. 3B ). Here, we measured a K D of 490 ± 368 n m for the Bs aptamer domain and 99 ± 38 n m for the Tt aptamer domain, respectively. Thus, there is good agreement for K D measurements between multiple different techniques. In addition to the selectivity measured by comparing different SMM screens (Fig. 1C ), we also used fluorescence titration to evaluate the binding of 1 to tRNA. Upon titrating tRNA into a solution of 1 , only non-specific binding was observed, and fluorescence quenching did not fit to a 1:1 binding model, indicating only weak binding to tRNA at high micromolar levels (Supplementary Fig. 3 ). Fig. 3 Affinity of 1 for PreQ 1 -RS aptamers. a Fluorescence intensity assay of 5′-Cy5-labeled Bs PreQ 1 -RS or 5′-AlexaFluor 647-labeled Tt PreQ 1 -RS RNA in the presence of increasing concentration of 1 . b Inherent fluorescence titration of 1 with increasing concentration of unlabeled Bs PreQ 1 -RS or Tt PreQ 1 -RS RNA. Error bars indicate the standard deviation determined from three independent measurements. Source data are provided as a Source Data file Full size image Ligand induces conformational change to riboswitch aptamers A key aspect of riboswitch biochemistry is that biological effects are driven by ligand-induced conformational changes in the RNA upon binding. Thus, we aimed to evaluate the effects of 1 on the conformation of the PreQ 1 aptamers by in-line probing experiments [30] . In-line probing experiments are routinely used to monitor alterations of riboswitch conformation and can report on ligand-induced effects on RNA structure. First, we performed in-line probing using a fluorescently tagged 36-mer Bs aptamer domain (5ʹ-AF647- Bs PreQ 1 -RS, Supplementary Table 1 ) with PreQ 1 . Consistent with previous reports using a radiolabeled 36-mer construct [30] , we observed an increase in cleavage at C12 and a corresponding decrease in cleavage at U32 (based on 34-mer numbering, Fig. 1D ). Thus, in-line probing using a fluorescently tagged construct accurately matches literature reports on ligand-induced conformational changes. Next, we performed an analogous experiment in the presence of synthetic ligand 1 (Fig. 4A ). In contrast to the cognate ligand, 1 caused an increase in cleavage at C8, U9, U13, C15, U22, and U24, whereas it did not induce prominent increase in cleavage at C12. Although these changes were consistent from experiment to experiment, smaller changes in cleavage at other residues (for example nucleotides 17–19) were less consistent from experiment to experiment and could not be attributed to a specific binding interaction. Thus, although the compound binds directly to the Bs aptamer domain and alters the conformation of the RNA, the effects of 1 in this assay are distinct from those of PreQ 1 . We also performed in-line probing with the Tt riboswitch (5ʹ-AF647- Tt PreQ 1 -RS, Supplementary Table 1 ). In this case, with PreQ 1 the most notable increase in cleavage occurred at U12 (Fig. 4B ). Upon addition of compound 1 , a similarly small increase in cleavage occurred at U12 and A13. Thus, 1 may induce a conformational change in the Tt aptamer similar to PreQ 1 . The Bs and Tt riboswitches have been previously described to have similar conformational ensembles but differ in their ability to recognize ligands by conformational selection and induced fit mechanisms, respectively [44] . This distinction may be reflected in the effects observed in in-line probing experiments. Fig. 4 Ligand-induced conformational changes. In-line probing of a 5′-AlexaFluor 647-labeled Bs PreQ 1 -RS RNA and b 5′-AlexaFluor 647-labeled Tt PreQ 1 -RS RNA after treatment with 1 at increasing concentrations or a DMSO control in the absence (–) or presence (+) of 1 m m MgCl 2 . Treatment with PreQ 1 at a concentration of 10 μ m is used as a positive control. OH and T1 are a partial alkaline hydrolysis ladder and ribonuclease T1 digestion, respectively. Arrows designate nucleotide positions where the cleavage efficiency was significantly altered by compound treatment (blue) or preQ 1 treatment (red) Full size image Ligand modulates riboswitch transcriptional termination Having demonstrated that 1 binds and causes conformational changes in both the Bs and Tt aptamers, we next evaluated 1 in a functional assay. As described above, the Bs riboswitch regulates the transcription of downstream genes upon ligand binding. Thus, we examined the capacity of 1 to modulate transcriptional termination. 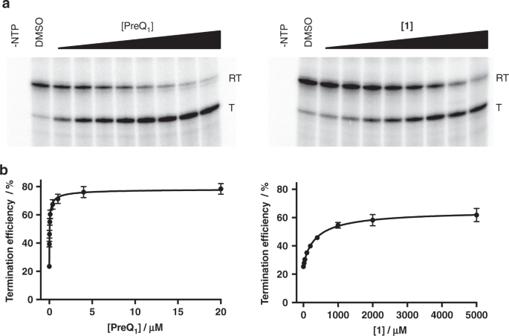Fig. 5 Transcription termination assay of1.aRepresentative gel images of the32P-labeled RNA products of in vitro transcription of theSsPreQ1-RS template in the presence of increasing concentrations of PreQ1(left) and1(right). Bands corresponding to the read-through transcription product (RT) and terminated transcription product (T) are indicated. Full gel images are provided in theSupplementary Information.bQuantification of transcription termination efficiency of increasing concentrations of PreQ1(left) or1(right). Error bars indicate standard deviation,n= 3. Source data are provided as a Source Data file DNA templates were designed containing the aptamer domain and terminator hairpin of the BsPreQ 1 riboswitch, followed by an elongation sequence (BsPreQ 1 TTA, Supplementary Table 5 ). In vitro transcription of these templates produces an RNA sequence containing the riboswitch. This transcription can either be halted at the terminator hairpin in the presence of the cognate ligand or produce a read-through product that is transcribed to the end of the template. Despite repeated attempts, efforts to observe transcriptional termination of the Bs riboswitch by PreQ 1 were unsuccessful in this assay. Staphylococcus saprophyticus ( Ss ) also contains a related PreQ 1 riboswitch sequence with a conserved binding site that functions by transcriptional termination (Fig. 1D ). Dose-dependent transcriptional termination was observed with a template containing the Ss riboswitch ( Ss PreQ 1 TTA, Supplementary Table 5 ). Near-complete termination was observed at the highest PreQ 1 concentrations tested with an EC 50 for PreQ 1 of 36 ± 5 n m (Fig. 5 ). Similarly, addition of increasing concentrations of 1 also resulted in near-complete termination of transcription with an EC 50 of 359 ± 23 μ μ . Thus, 1 functions by a mechanism similar to PreQ 1 itself. We also confirmed that 1 binds to the Ss aptamer by WaterLOGSY experiments (Supplementary Fig. 4 ). In addition, the K D of 1 for the Ss aptamer was determined to be by 42 ± 6 n m by fluorescence titration (Supplementary Fig. 5 ). As a further control, the chemically unrelated ligand 5-aminoimidazole-4-carboxamide ribonucleotide, which binds to other riboswitches [47] , was tested in transcriptional assays and had no effect on the Ss reporter construct (Supplementary Fig. 7 ). Fig. 5 Transcription termination assay of 1 . a Representative gel images of the 32 P-labeled RNA products of in vitro transcription of the Ss PreQ 1 -RS template in the presence of increasing concentrations of PreQ 1 (left) and 1 (right). Bands corresponding to the read-through transcription product (RT) and terminated transcription product (T) are indicated. Full gel images are provided in the Supplementary Information . b Quantification of transcription termination efficiency of increasing concentrations of PreQ 1 (left) or 1 (right). Error bars indicate standard deviation, n = 3. Source data are provided as a Source Data file Full size image X-Ray crystal structure of the ligand/aptamer complex To establish a molecular basis for its selective binding, we solved crystal structures of 1 bound to the Tt PreQ 1 riboswitch aptamer domain. Initial efforts using the wild-type Tt PreQ 1 riboswitch aptamer domain failed, yielding structures indistinguishable from the previously reported ligand-free aptamer domain structure of the RNA, in which the nucleobase of A14 occupies the PreQ 1 -binding site [29] . To alleviate competition by the intramolecular interaction with binding of the exogenous ligand, we designed aptamer domains in which the nucleobase at position 14, as well as one or two adjacent disordered loop nucleobases were removed. (ab13_14 and ab13_14_15, Supplementary Table 1 ). Co-crystal structures of these abasic Tt PreQ 1 riboswitch aptamer domains complexed with 1 (ab13_14- 1 , and ab13_14_15- 1 ) were determined by the molecular replacement (MR) method and both refined at 1.8 Å resolution. These two structures are near-identical (r.m.s.d. is 0.14 Å for 638 non-hydrogen atom pairs). The following discussion focuses on the ab13_14- 1 complex. We also determined the crystal structure of ab13_14 in complex with PreQ 1 (ab13_14-PreQ 1 ) at 1.69 Å resolution, for comparison (Methods and Supplementary Table 7 ). 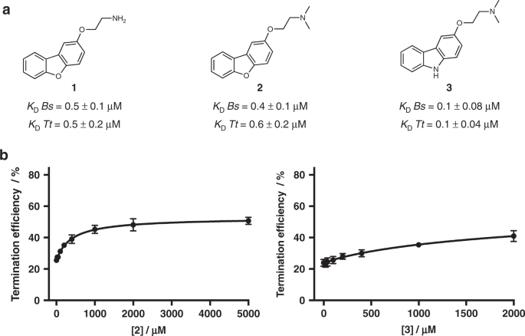Fig. 7 Evaluation of modified analogs of2and3.aApparentKDvalues for1–3as determined by fluorescence intensity assays with 5′-Cy5-BsPreQ1-RS and 5′-AlexaFluor 647-TtPreQ1-RS RNA. Values are the mean ± s.d. (error bars) of three replicate measurements.bQuantification of termination efficiency of increasing concentrations of2(left) and3(right) in transcription termination assays of a DNA template containing theSsPreQ1riboswitch. Error bars indicate the standard deviation determined from three independent measurements. Source data are provided as a Source Data file. Gel images are provided in theSupplementary Information Unbiased | F o |−| F c | residual electron-density maps unambiguously located 1 at the interhelical interface of stems S1 and S2, surrounded by the L2 and L3 loops, in both co-crystal structures (Fig. 6A , ab13_14- 1 ; Supplementary Fig. 8 , ab13_14_15- 1 ). Thus, the synthetic ligand occupies a position similar to that of the cognate ligand PreQ 1 . The dibenzofuran of 1 is sandwiched between G11 and the G5•C16 pair, with the furan oxygen engaging in a hydrogen bond (3.2 Å) with the N6 atom of A29 (Fig. 6B and Supplementary Fig. 5 ). The same oxygen is in van der Waals contact with the N1 atom of A29 (3.7 Å) The nucleotides that interact with 1 are phylogenetically conserved among PreQ 1 riboswitches (Fig. 1D ), being responsible for PreQ 1 recognition (Supplementary Fig. 9 ) [28] . In contrast to the solvent-inaccessible heterocycle of 1 , its amine-bearing sidechain (largely coplanar with the dibenzofuran heterocycle) is solvent exposed, with the amine hydrogen bonding to water, and therefore not directly recognized by the RNA (Fig. 6B ). However, to avoid steric clash with the L2 loop, 1 must bind with its sidechain emerging from the PreQ 1 -binding pocket away from L2 loop of the riboswitch. Of note, lack of direct recognition of the amine of 1 provides a plausible explanation for how the binding event occurred when 1 was chemically conjugated to the SMM slide. Although the sugar of residue 13 of the ab13_14- 1 structure lacked electron density and is presumed disordered, in the ab13_14_15- 1 structure, the ribose ring of residue 13 is ordered and in van der Waals contact with ring C of the dibenzofuran of 1 (Supplementary Figure 8 ). 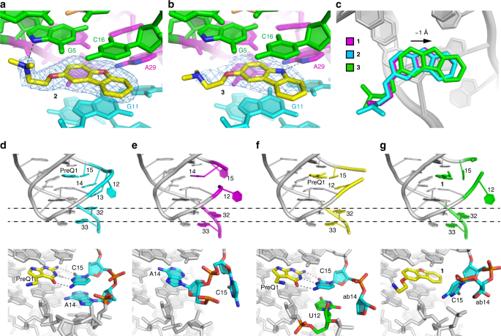Fig. 8 Structural analysis of the boundTtPreQ1aptamers.aLigand-binding site of the ab13_14-2co-crystal structure, superimposed on the |Fo|−|Fc| electron-density map calculated before addition of the ligand to the crystallographic model (blue mesh, 3.0 σ contour). Hydrogen bonds are indicated as dotted lines.bLigand-binding site of the ab13_14_15-3co-crystal structure. The |Fo|−|Fc| electron density map for the compound is colored blue and contoured at 3.0 σ.cComparison of binding modes of1(magenta),2(cyan), and3(green). Ligand-binding site and continuous base stack of the aptamer domains of thedWT-PreQ1,eWT free,fab13_14-PreQ1, andgab13_14-1forms. (Upper) Cartoon representations with ligands and key nucleotides labeled and colored cyan, magenta, yellow, and green in the WT-PreQ1, WT free, ab13_14-PreQ1, and ab13_14-1forms, respectively. To compare the locations of A32 and G33 among these structures, dashed lines are indicated. (Lower) Detail of the ligand-binding site. PreQ1and1are in yellow. Key nucleotides responsible for forming the base stack are colored cyan. U12 in the ab13_14-PreQ1structure, which occupies a similar location to A14 in the WT-PreQ1structure, is in green. Hydrogen bonds between PreQ1and C15 are indicated as dotted lines Fig. 6 Co-crystal structure of the aptamer complexed with 1 . a Overall structure of the complex. S1, S2, L1, L2, and L3 are colored green, cyan, magenta, gray, and orange, respectively. The nucleotides between L3 and S2, which interact with L1, are also in magenta. Unbiased | F o |−| F c | electron density map for the compound 1 (blue mesh) contoured at 3.0 σ. b Detail of the ligand-binding site. Nucleotides that interact with 1 are labeled. Dotted lines denote hydrogen bonds between 1 and a bound water molecule and with A29 Full size image Structure-guided changes alter mode of binding and activity Next, we asked whether alteration of the chemical structure of 1 would have effects on riboswitch recognition or activity. We hypothesized that alteration of the basicity of the pendant amine of 1 might enable it to engage in hydrogen-bonding contacts with the RNA. Thus, we prepared the dimethylamino derivative 2 , containing a more basic tertiary amine (Fig. 7A ). We evaluated the affinity of 2 for both the Bs and Tt aptamers by monitoring changes in fluorescence of the 5ʹ-Cy5- Bs PreQ 1 -RS and 5ʹ-AF647- Tt PreQ 1 -RS RNAs (Supplementary Table 1 ) upon titration with 2 and determined affinities of 0.4 ± 0.1 μ m and 0.6 ± 0.2 μ m , respectively (Supplementary Fig. 10 ). In addition to the pendant amine, we asked whether alteration of the core heterocyclic scaffold would have effects on RNA binding. We noted that in the structure of 1 bound to the riboswitch, the exocyclic amine of A29 makes a hydrogen bond with the oxygen atom of the dibenzofuran. In this structure, A29 is not coplanar with 1 and sits at an angle of 40°, where N1 and N6 bisect the plane of the dibenzofuran core. Nucleotides are amphiphilic and are capable of serving as both hydrogen bond donors and acceptors. We therefore synthesized a carbazole derivative of 2 , compound 3 (Fig. 7A ), replacing the dibenzofuran oxygen with a nitrogen atom (that may potentially donate a hydrogen bond). Affinities of 3 for the Bs and Tt riboswitch aptamer domains were measured to be 0.1 ± 0.08 μ m and 0.1 ± 0.04 μ m , respectively, using fluorescence titrations (Supplementary Fig. 10 ). Thus, all three compounds have similar affinities for the riboswitch aptamers. Finally, 2 and 3 were evaluated in transcriptional termination assays (Fig. 7B , Supplementary Fig. 11 ). Here, 2 behaved similarly to 1 in terms of maximal effect. However, 3 was markedly inferior in the functional assay. Fig. 7 Evaluation of modified analogs of 2 and 3 . a Apparent K D values for 1 – 3 as determined by fluorescence intensity assays with 5′-Cy5- Bs PreQ 1 -RS and 5′-AlexaFluor 647- Tt PreQ 1 -RS RNA. Values are the mean ± s.d. (error bars) of three replicate measurements. b Quantification of termination efficiency of increasing concentrations of 2 (left) and 3 (right) in transcription termination assays of a DNA template containing the Ss PreQ 1 riboswitch. Error bars indicate the standard deviation determined from three independent measurements. Source data are provided as a Source Data file. Gel images are provided in the Supplementary Information Full size image To further understand the interactions of 2 and 3 with the riboswitches, we also solved crystal structures of each ligand in complex with the Tt riboswitch. The co-crystal structures of abasic mutant riboswitch aptamer domains bound to 2 and 3 (ab13_14- 2 and ab13_14_15- 3 , respectively) were solved by the MR method and refined at 1.94 Å and 2.56 Å resolution, respectively (Methods and Supplementary Table 7 ). The overall structure of ab13_14- 2 is similar to that of the riboswitch bound to 1 , with 2 in a similar binding pose, directly in the PreQ 1 binding site (Fig. 8A ). In this structure, the sidechain of 2 bends upwards at the methylene preceding the amine, bringing the pyramidal tertiary amine of 2 within hydrogen-bonding distance (2.9 Å) of the N7 atom of the phylogenetically conserved G5 of the riboswitch (Fig. 1D ). In contrast, the primary amine of 1 lies 3.6 Å from the same RNA atom. Next, we solved the crystal structure of 3 in complex with the Tt riboswitch aptamer domain. Similar to 1 and 2 , compound 3 occupies the PreQ 1 -binding site (Fig. 8B ). However, in this structure, 3 has shifted by ~1 Å in the direction of RNA loop L2 (Fig. 8C ) to support a hydrogen bond between the new donor atom in the heterocycle and the RNA (the distances between the carbazole nitrogen atom of 3 and the N1 and N6 atoms of A29 are 3.2 Å and 3.5 Å, respectively). This confirms that alteration of the chemical structure of the initial hit can lead to changes in binding modes and somewhat altered affinity. Possibly owing to the ~1 Å shift in its binding pose (Fig. 8C ), the conformation of the sidechain of the bound 3 resembles that of the bound 1 rather than that of 2 . The sidechain of the bound 3 is largely coplanar with the carbazole, exposed to solvent, and does not lie within hydrogen-bonding distance of G5 of the RNA. Fig. 8 Structural analysis of the bound Tt PreQ 1 aptamers. a Ligand-binding site of the ab13_14- 2 co-crystal structure, superimposed on the | F o |−| F c | electron-density map calculated before addition of the ligand to the crystallographic model (blue mesh, 3.0 σ contour). Hydrogen bonds are indicated as dotted lines. b Ligand-binding site of the ab13_14_15- 3 co-crystal structure. The | F o |−| F c | electron density map for the compound is colored blue and contoured at 3.0 σ. c Comparison of binding modes of 1 (magenta), 2 (cyan), and 3 (green). Ligand-binding site and continuous base stack of the aptamer domains of the d WT-PreQ 1 , e WT free, f ab13_14-PreQ 1 , and g ab13_14- 1 forms. (Upper) Cartoon representations with ligands and key nucleotides labeled and colored cyan, magenta, yellow, and green in the WT-PreQ 1 , WT free, ab13_14-PreQ 1 , and ab13_14- 1 forms, respectively. To compare the locations of A32 and G33 among these structures, dashed lines are indicated. (Lower) Detail of the ligand-binding site. PreQ 1 and 1 are in yellow. Key nucleotides responsible for forming the base stack are colored cyan. U12 in the ab13_14-PreQ 1 structure, which occupies a similar location to A14 in the WT-PreQ 1 structure, is in green. Hydrogen bonds between PreQ 1 and C15 are indicated as dotted lines Full size image In this work, we report the discovery of synthetic ligands that bind to different PreQ 1 riboswitch aptamer domains. Compounds discussed here are characterized by multiple orthogonal biophysical techniques, and exhibit submicromolar dissociation constants to the RNA. Furthermore, structural probing experiments indicate clear ligand-induced conformational changes. As a consequence of binding, the compounds exhibit activity in transcriptional termination assays, inducing premature termination analogous to those produced by the cognate ligand itself. Thus, the compounds function by a mechanism similar to PreQ 1 , despite having no obvious chemical similarity. Structural characterization of the ligand-aptamer complexes by X-ray crystallography provides insights into both the mode of recognition and mechanism of action of these compounds. Structural comparison between ab13_14- 1 and the PreQ 1 -bound wild-type Tt PreQ 1 riboswitch (referred to as WT-PreQ 1 ) reveals conformational differences in four nucleotides (positions 12–15) of the L2 loop and two nucleotides at the 3’-end (A32 and G33) of these complexes. In the WT-PreQ 1 structure, C15 recognizes PreQ 1 through Watson-Crick base pairing and serves as a starting point of the consecutive base stack, C15-A14-A13-A32-G33. The last two nucleotides (A32 and G33) of the base stack constitute the Shine-Dalgarno sequence and form stem S2 by base-pairing with A10 and C9, respectively. Therefore, the continuous base stack is proposed to be crucial to inhibit gene expression through sequestrating the Shine-Dalgarno sequence from the recognition by the ribosome. Because 1 is bulkier than PreQ 1 , compound-binding interferes with the correct positioning of C15. Consequently, C15 in the ab13_14- 1 structure shifts position and its base is placed perpendicular to that of the WT-PreQ 1 structure to escape the steric clash with 1 (Fig. 8 D and G ). Moreover, A32 and G33 are located downward (far away from ligand binding site) compared to those of the WT-PreQ 1 structure. Therefore, the ab13_14- 1 structure is similar to the free state of the riboswitch, despite the difference that the ligand-binding site was occupied by A14 in the latter structure (Fig. 8 E and G ). The striking contrast between the ab13_14- 1 and WT-PreQ 1 structures is predominantly attributable to the binding of the bulkier compound to the riboswitch. Consistent with this, the crystal structure of ab13_14-PreQ 1 showed a similar conformation to WT-PreQ 1 rather than ab13_14- 1 , where C15 in ab13_14-PreQ 1 is well superimposed to that in WT-PreQ 1 and A32 and G33 in ab13_14-PreQ 1 shift toward the ligand-binding site compared with the ab13_14- 1 structure (Fig. 8D–G and Supplementary Fig. 5 ). In addition, U12 of ab13_14-PreQ 1 is placed in a similar location to A14 of WT-PreQ 1 and hydrogen bonds with G11 in order to compensate for the absence of the base at position 14. Therefore, PreQ 1 binding to the ligand binding site results in a conformation similar to WT-PreQ 1 despite the absence of the bases at positions 13 and 14. From these findings, 1 binding to the wild-type Tt PreQ 1 riboswitch may induce a suboptimal formation of the continuous base stack that transmits the ligand binding information to the expression platform of the riboswitch. This suboptimal conformation may lead to the decreased maximum termination efficiency in the transcription termination assay for 1 in comparison with the cognate ligand. Like the translational class I PreQ 1 riboswitch, transcriptional class I PreQ 1 riboswitches also have a continuous base stack from the ligand-binding site to the expression platform. Given that the transcriptional and translational PreQ 1 riboswitches control ON/OFF switching using similar structural motifs, the 1 -bound Tt PreQ 1 riboswitch structure can explain why this compound has an EC 50 of 359 ± 23 μ m in transcription termination assays ( Ss aptamer). This value is considerably higher than that for PreQ 1 (36 ± 5 n m ) despite affinities of 0.5 ± 0.1 μ m and 4 ± 0.6 n m , respectively ( Bs aptamer). These findings suggest that the region of 1 situated near C15 would be a good candidate for synthetic efforts to improve the potency for downregulating gene expression. Our co-crystal structures are the starting point for developing additional compounds that target the bacteria-specific Q biosynthetic pathway. Although 1 , 2 , and 3 have similar binding affinities for the Tt and Bs aptamers, they do not have identical activity in transcription termination with the Ss riboswitch. This difference in activity may be due to subtle differences in binding modes to the RNA, reflected in the lack of a hydrogen bond to G5 and the altered pose of ligand 3 . Importantly, the synthetic ligand has considerably decreased solubility at concentrations needed for transcription termination, which may also play a role in decreased function. Although it has been previously demonstrated that binding affinity is not the sole parameter that governs the activity of RNA-binding compounds [48] , these observations are often not accompanied by mechanistic or structural rationalization. Our work demonstrates that subtle alterations in the mode of recognition of ligands may also have a role in the ability of a compound to induce conformational or functional effects. This work highlights a challenge in developing ligands for functional RNAs, namely that affinity is not the only property that governs the activity of a compound. Finally, the work described herein illustrates the role structure has in understanding the behavior of small synthetic compounds that bind to and modulate the function of complex RNAs. General RNA methods To avoid RNase contamination, all buffers were prepared with diethyl pyrocarbonate-treated water and all surfaces and equipment were decontaminated with RNaseZap (Ambion) prior to RNA handling. Deprotected and high-performance liquid chromatography purified oligonucleotides were purchased from Dharmacon (ThermoFisher) or IDT DNA. Sequences of the RNA oligonucleotides used for biochemical and biophysical experiments can be found in Supplementary Table 1 . SMM screening SMM slides were prepared according to established procedures [36] , [38] . In brief, γ-aminopropyl silane microscope slides (Corning) were functionalized with an Fmoc-protected amino polyethylene glycol spacer (Fmoc-8-amino-3,6-dioxaoctanoic acid) in N,N -dimethylformamide (DMF). Following piperidine deprotection, 1,6-diisocyanatohexane was coupled to the surface to provide isocyanate-functionalized microarray slides for immobilization of small molecule library members. A total of 26,227 small molecules (10 m m in DMSO) containing at least one primary or secondary alcohol or amine were purchased from commercial vendors including ChemBridge and ChemDiv. The libraries were printed on seven array slides containing ~ 3840 distinct molecules printed in duplicate, in addition to dyes and controls used for quality-control validation. The arrays were exposed to pyridine vapor to facilitate covalent attachment to the isocyanate-functionalized slides. Slides were then incubated with a 1:20 polyethylene glycol:DMF (v/v) solution to quench unreacted isocyanates. The 5′-Cy5- Bs PreQ 1 -RS RNA was dissolved in 50 m m Tris, 100 m m KCl, 1 m m MgCl 2 , pH 7.5, diluted to 5 µ m , and was annealed by heating to 75 °C for 5 min, followed by slowly cooling to room temperature for 30 min. The annealed RNA was then further diluted to 1 µ m in 50 m m Tris, 100 m m KCl, 1 m m MgCl 2 , pH 7.5 for screening. Printed microarray slides were incubated with the RNA at a concentration of 1 µ m for 2 h using a LifterSlip (Electron Microscopy Sciences). Following incubation, slides were washed three times with 4 mL of 50 m m Tris, 100 m m KCl, 1 m m MgCl 2 , pH 7.5 buffer for 2 min in a four-well Nunc plate, and the slides were dried by centrifugation for 2 min at 4000 × g. Slides were imaged for fluorescence (650 nm excitation, 670 nm emission) on an Innopsys Innoscan 1100 AL Microarray Scanner with a resolution of 5 μm. The scanned image was aligned with the corresponding GenePix Array List (GAL) file to identify individual features. Hits were determined based on signal-to-noise ratio (SNR), defined as (mean foreground−mean background)/standard deviation of background, and Z -score, defined as: Z = (Mean SNR635compound—Mean SNR635library)/(SD SNR635library) with the following criteria: (a) coefficient of variance of duplicate spots < 100, (b) Average Z-score for a compound > 3, (c) [( Z -score RNA incubated )—( Z -score Control Array )]/ Z -score Control Array ) > 3, (d) no activity with any other nucleic acid structures screened in parallel. Other Cy5-labeled riboswitches screened in parallel included TPP and SAM-II, which were screened using the same method described above for the PreQ 1 riboswitch. Hits were further validated by visual inspection of array images and compounds for further study were purchased from original suppliers. General ligand observed NMR methods All NMR spectra were recorded at 293 K on a Bruker AVANCE III 500 MHz spectrometer equipped with a TCI cryoprobe. NMR buffer was composed of 50 m m Tris- d 11 , pH 7.5, 100 m m KCl, 1 m m MgCl 2 in 100% UltraPure distilled H 2 O (Invitrogen). Subsequently prepared NMR samples contained 10% D 2 O and 5% DMSO- d 6 to improve compound solubility. All compounds were first dissolved to a 10 m m stock concentration in 100% DMSO- d 6 prior to NMR sample preparation. Purchased RNA was buffer exchanged (3 kDa MWCO spin column, EMD Millipore) into the NMR buffer prior to use. For WaterLOGSY and CPMG experiments, a reference 1D- 1 H spectrum was collected for each sample using the “zgesgp” excitation sculpting water suppression pulse sequence from Bruker, with 128 scans. All data was processed and visualized with MestReNova software (Version 8.1.2-11880). WaterLOGSY NMR Bs PreQ 1 -RS and Tt PreQ 1 -RS RNA were buffer exchanged into 50 m m Tris- d 11 , pH 7.5, 100 m m KCl, 1 m m MgCl 2 in UltraPure distilled H 2 O using centrifugal filtration (3 kDa MWCO, EMD Millipore) and were annealed by heating to 75 °C for 5 min, followed by slowly cooling to room temperature for 30 min. NMR samples containing each SMM compound at a concentration of 375 µ m and a negative control N -methyl- l -valine (Chem-Impex-International) at 375 µ m were prepared in 50 m m Tris- d 11 , pH 7.5, 100 m m KCl, 1 m m MgCl 2 in UltraPure distilled H 2 O containing 10% D 2 O and a final concentration of 5% DMSO- d 6 . For each compound, samples were prepared with and without each RNA at a concentration of 15 µ m . Samples were incubated on ice for 10 min, degassed at 20 °C for 15 min, and transferred to a Shigemi NMR tube. A reference 1D- 1 H and 1D WaterLOGSY spectra with and without RNA were recorded. NMR spectra were recorded at 293 K on a Bruker AVANCE III 500 MHz spectrometer equipped with TCI cryoprobe [43] . CPMG NMR Bs PreQ 1 -RS and Tt PreQ 1 -RS RNA were buffer exchanged into 50 m m Tris- d 11 , pH 7.5, 100 m m KCl, 1 m m MgCl 2 in UltraPure distilled H 2 O using centrifugal filtration (3 kDa MWCO, EMD Millipore) and were annealed by heating to 75 °C for 5 min, followed by slowly cooling to room temperature for 30 min. Samples of 1 (300 μ m ) with or without each RNA (3 μ m ) were prepared in 50 m m Tris- d 11 , pH 7.5, 100 m m KCl, 1 m m MgCl 2 in UltraPure distilled H 2 O containing N -methyl- l -valine (300 μ m ), 10% D 2 O, and 5% DMSO- d 6 . Samples were incubated on ice for 10 min, degassed at 20 °C for 15 min, and transferred to a Shigemi NMR tube. NMR spectra were acquired at 298 K on a Bruker AVANCE III 500 MHz spectrometer fitted with a TCI Cryoprobe with Z-gradient. CPMG data sets with Presaturation Water Suppression (cpmgpr1d) were acquired using a 200 ms T 2 relaxation filter (d 2 0=0.001 s, L4=200) with a 10-second relaxation delay. O1 was set to 2349.67 Hz, RG to 203, and data sets were acquired with 64 scans. The spectra of the sample with and without RNA were aligned and scaled so that the peak heights of the internal standard N -methyl- l -valine were equivalent. Significantly attenuated ligand peaks (≥ 20%) in the presence of RNA were considered indicative of small molecule binding [45] . Fluorescence intensity assay Fluorescence titrations were performed using either a 5′-Cy5- Bs PreQ1-RS or AF647- Tt PreQ1-RS. Each RNA was diluted into 50 m m Tris, 100 m m KCl, 1 m m MgCl 2 , pH 7.5 to a concentration of 10 µ m and was annealed by heating to 75 °C for 5 min, followed by slowly cooling to room temperature for 30 min. Small molecule solutions were prepared as serial dilutions in 10% DMSO in buffer. In a cuvette, RNA was diluted to a final concentration of 50 n m in 50 m m Tris, 100 m m KCl, 1 m m MgCl 2 , pH 7.5 buffer containing 10% DMSO. Small molecules were titrated to final concentrations ranging from 0 to 77.4 μ m maintaining a 10% final DMSO concentration. After delivery of the small molecule, the sample was allowed to equilibrate for 8 min at room temperature. The fluorescence emission spectrum was then measured at room temperature using a Photon Technology International, Inc. QuantaMaster 600 TM Spectrofluorometer equipped with Felix GX 4.2.2 software. Fluorescence was recorded at an excitation wavelength of 649 nm and an emission of 655–800 nm. Total area under the peak from 655–700 nm was quantified and was then normalized to the values obtained for RNA incubated with a DMSO control. Normalized fluorescence for three independent replicates were averaged and plotted against small molecule concentration. K D values were determined using a single site-binding model. Inherent ligand fluorescence titration Fluorescence titrations were performed using either unlabeled Bs PreQ1-RS or Tt PreQ 1 -RS. Each RNA was resuspended to a concentration of ~ 500 µ m in 50 m m Tris, pH 7.5, 100 m m KCl, 1 m m MgCl 2 , and annealed by heating to 75 °C for 5 min, followed by slowly cooling to room temperature for 30 min. Serial dilutions of each RNA were prepared in 50 m m Tris, pH 7.5, 100 m m KCl, 1 m m MgCl 2 . Inherent fluorescence titrations were performed with compound 1 at a final concentration of 500 n m in 50 m m Tris, pH 7.5, 100 m m KCl, 1 m m MgCl 2 with 5% DMSO. For Bs PreQ 1 -RS, in a black 384-well plate, 1 was diluted to a final concentration of 500 n m in buffer with a 5% final DMSO concentration. RNA was added to final concentrations ranging from 0–50 μ m in triplicate, the plate was centrifuged (1000 rpm, 2 min), and samples were allowed to incubate for 30 min at room temperature with shaking. The fluorescence intensity was then measured on a Synergy Mx microplate reader (BioTek) at an excitation wavelength of 300 nm and an emission wavelength of 340 nm (gain = 120). The fluorescence intensity was then normalized to the values obtained for 1 in the absence of RNA and was plotted against RNA concentration. The dissociation constants were determined using a single site binding model. For Tt PreQ 1 -RS, in a cuvette, 1 was diluted to a final concentration of 500 n m in 50 m m Tris, pH 7.5, 100 m m KCl, 1 m m MgCl 2 buffer with a 5% final DMSO concentration. RNA was titrated to final concentrations ranging from 0 to 7 μ m and the sample was allowed to equilibrate for 8 min at room temperature after each addition. The fluorescence emission spectrum was then measured at room temperature using a Photon Technology International, Inc. QuantaMaster 600 TM Spectrofluorometer equipped with Felix GX 4.2.2 software. Fluorescence was recorded at an excitation wavelength of 300 nm and an emission of 320-460 nm. Total area under the peak from 320-380 nm was quantified and was then normalized to the values obtained for 1 in the absence of RNA. Normalized fluorescence for three independent replicates were averaged and plotted against RNA concentration. K D values were determined using a single site binding model. Analysis of Mg 2+ -induced in-line cleavage This procedure was adapted from a related procedure that used radiolabeled oligonucleotides [30] . 5′-AF647- Bs PreQ 1 -RS or 5′-AF647- Tt PreQ 1 -RS RNA was diluted into 50 m m Tris, 100 m m KCl, pH 7.5 to a concentration of 10 µ m and were annealed by heating to 75 °C for 5 min, followed by cooling on ice for 10 min. The annealed RNA was incubated at a final concentration of 1 μ m in 50 m m Tris, pH 8.3, 10 m m KCl buffer with either a DMSO control (5% final concentration) or compound 1 at a concentration of 0.1, 1, 3, 10, 30, 100, or 300 μ m . For 5′-AF647- Bs PreQ 1 -RS, MgCl 2 was added at a final concentration of 2 m m , and the reactions were incubated at room temperature in darkness for 40 hrs. For 5′-AF647- Tt PreQ 1 -RS, MgCl 2 was added at a final concentration of 2 m m , and the reactions were incubated at room temperature in darkness for 72 h to reach the desired level of cleavage. Alkaline hydrolysis was performed in 50 m m NaHCO 3 , pH 9.0 at 95 °C for 5 min. Ribonuclease T1 digestion was carried out with 0.1 U of ribonuclease T1 (Ambion) in 20 m m Tris, pH 7.5, 50 m m NaCl, 0.1 m m MgCl 2 at room temperature for 20 min. The RNase T1 reaction was stopped by adding 0.2 volumes of 5 m m EDTA. Equal volumes of loading buffer containing 7 m urea, 1 × Tris-borate-EDTA (TBE), and 0.01% direct red dye was added to each reaction, and the samples were heated to 95 °C for 5 min. 10 µL of each sample was analyzed by electrophoresis on a denaturing polyacrylamide sequencing gel (20% polyacrylamide, 19:1 crosslinking, 7 m urea) at 60 W, 45 °C for 3.5 hrs. The gel was visualized by fluorescence of the 5′-Cy5 label (630 nm excitation, 670 emission) with Typhoon FLA 9500 Phosphorimager (GE Healthcare Life Sciences) and was analyzed with ImageQuant software. X-ray crystallography RNA preparation Sequences of the RNAs employed in this study are based on Tt PreQ1 riboswitch aptamer domain and listed in Supplementary Table 1 . RNAs were purchased from Dharmacon and deprotected according to the manufacturer’s instructions. After lyophilization, RNAs were dissolved in water and stored at − 25 °C. Crystallization and diffraction data collection RNA solutions containing 11.8 m m sodium cacodylate (pH 7.0) were heated at 65 °C for 2 min. MgCl 2 and synthetic compound were then added to the final concentrations of 10 m m and 0.5 m m , respectively. The solutions were incubated at 65 °C for 3 min, and then cooled down gradually to the room temperature. Tt PreQ 1 riboswitch was crystallized by the hanging-drop vapor diffusion method at 21 °C, under conditions containing 5–15 m m Mg acetate, 50 m m MES (pH 5.6), and 2.3–2.7 m ammonium sulfate (Condition I) and containing 0.1–0.3 m potassium sodium tartrate, 100 m m sodium citrate (pH 5.6), and 2.0–2.8 m ammonium sulfate (Condition II). Hanging drops were prepared by mixing 1 μL of the RNA solution (0.38 m m RNA in 10 m m sodium cacodylate, pH 7.0, 10 m m MgCl 2 , and 0.5 m m synthetic compound) with 1 μL of the reservoir solution and were equilibrated against 400 μL of reservoir solution. The RNA crystals grew within 2 weeks to maximum dimensions of 300 × 100 × 100 μm 3 . For data collection, the RNA crystals were transferred to the cryoprotectant solutions containing 10 m m Mg acetate, 27.5 m m MES (pH 5.6), and 2.15 M lithium sulfate for the crystals obtained with the Condition I, and 60 m m potassium sodium tartrate, 25 m m sodium citrate (pH 5.6), and 2.15 M lithium sulfate for the crystals under the Condition II. The crystals were mounted in a nylon loop and flash frozen by plunging into liquid nitrogen. X-ray diffraction data were collected at the beamlines 5.0.1 and 5.0.2 of the Advanced Light Source (ALS), Lawrence Berkeley National Laboratory. Diffraction data were integrated and scaled with the program DIALS [49] . Data processing statistics are summarized in Supplementary Table 7 . Structure determination and refinement The structures were solved by the MR method using the previously determined T. tengcongensis PreQ 1 aptamer structure (PDB ID: 3Q51 [ https://doi.org/10.2210/pdb3Q51/pdb ]) as a search model with the program PHASER [50] . The solutions were subjected to simulated annealing, energy minimization, restrained isotropic B-factor, and TLS refinement with PHENIX [51] , and the resulting electron-density maps revealed the locations of the small molecules. Iterative cycles of refinement and manual rebuilding [52] produced the current co-crystal structures of ab13_14- 1 , ab13_14_15- 1 , ab13_14- 2 , ab13_14_15- 3 , and ab13_14-PreQ 1 with R free of 20.5, 20.5, 20.3, 24.8, and 21.0% at 1.80, 1.80, 1.94, 2.56, and 1.69 Å resolution, respectively. Refinement statistics are summarized in Supplementary Table 7 . Molecular graphics were produced with PyMol (http://www.pymol.org/). Stereo images are provided in Supplementary Figure 12 and 13 . 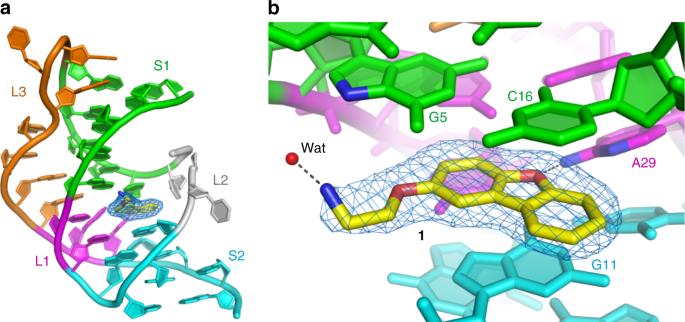Single-round transcription termination assay The transcription termination assays were carried out according to established protocols [53] , [54] with several modifications. The DNA plasmid containing λ PR promoter and 26-nt C-less sequence followed by the Staphylococcus saprophyticus PreQ 1 riboswitch and its downstream sequence cloned into pIDTSMART-AMP was purchased from Integrated DNA Technologies. Fig. 6 Co-crystal structure of the aptamer complexed with1.aOverall structure of the complex. S1, S2, L1, L2, and L3 are colored green, cyan, magenta, gray, and orange, respectively. The nucleotides between L3 and S2, which interact with L1, are also in magenta. Unbiased |Fo|−|Fc| electron density map for the compound1(blue mesh) contoured at 3.0 σ.bDetail of the ligand-binding site. Nucleotides that interact with1are labeled. Dotted lines denote hydrogen bonds between1and a bound water molecule and with A29 The DNA template was amplified by PCR from the plasmid using forward and reverse primers (Supplementary Table 6 ), and then was gel-extracted after agarose gel electrophoresis for purification. Halted transcription complexes were prepared in a solution containing 1 µ m GTP, 5 µ m ATP, 5 µ m UTP, 100 µ m ApU, [α- 32 P] GTP, 75 n m DNA template, 0.0167 U/µL Escherichia coli RNA polymerase holoenzyme (New England BioLabs) in 1 × transcription buffer (20 m m Tris-HCl, pH 8.0, 2 m m NaCl, 1 m m MgCl 2 , 4% glycerol, 0.1 m m DTT, and 0.1 m m EDTA), and incubated at 37 °C for 15 min. A DNA oligonucleotide complementary to the 26-nt C-less sequence was added to the reactions at 1.1 µ m final concentration in 1 × transcription buffer and incubated at room temperature for 5 min, in order to prevent undesired non-specific interactions between the 26-nt C-less sequence and riboswitch. Elongation was restarted by combining 9 µL of halted transcription complex, 3 µL of the compound (0–25 m m compound and 25% DMSO in 1 × transcription buffer), and 3 µL of NTPs mix (200 µ m ATP, 200 µ m CTP, 200 µ m GTP, 200 µ m UTP, 100 µg/mL heparin, and 250 m m KCl in 1 × transcription buffer), and incubated at 37 °C for 20 min. To remove the DNA template, 0.5 U of RQ1 RNase-Free DNase (Promega) was added to the reactions and incubated at 37 °C for 10 min. The reactions were stopped by adding equal volume of loading dye (8 m urea, 20% sucrose, 0.05% bromophenol blue, and 0.05% xylene cyanol in 2 × TBE). The reaction mixture was separated by 8% denaturing PAGE and visualized by phosphorimager. Full gel images are provided as Supplementary Figures. The band intensity was analyzed by ImageQuant software (GE Healthcare). Termination efficiency was calculated with dividing the intensity for the terminated RNA band by those for the total (terminated and antiterminated) RNAs. The sequences of the DNA oligonucleotides used in the transcription termination assay are summarized in Supplementary Table 5 . Synthetic procedures and characterization Chemical synthesis and compound characterization are provided in the Supplementary Methods . Reporting summary Further information on experimental design is available in the Nature Research Reporting Summary linked to this article.